MicroRNA122 is a key regulator of α-fetoprotein expression and influences the aggressiveness of hepatocellular carcinoma α-fetoprotein (AFP) is not only a widely used biomarker in hepatocellular carcinoma (HCC) surveillance, but is also clinically recognized as linked with aggressive tumour behaviour. Here we show that deregulation of microRNA122, a liver-specific microRNA, is a cause of both AFP elevation and a more biologically aggressive phenotype in HCC. We identify CUX1, a direct target of microRNA122, as a common central mediator of these two effects. Using liver tissues from transgenic mice in which microRNA122 is functionally silenced, an orthotopic xenograft tumour model, and human clinical samples, we further demonstrate that a microRNA122/CUX1/microRNA214/ZBTB20 pathway regulates AFP expression. We also show that the microRNA122/CUX1/RhoA pathway regulates the aggressive characteristics of tumours. We conclude that microRNA122 and associated signalling proteins may represent viable therapeutic targets, and that serum AFP levels in HCC patients may be a surrogate marker for deregulated intracellular microRNA122 signalling pathways in HCC tissues. The incidence of hepatocellular carcinoma (HCC), the third most common cause of cancer-related mortality worldwide [1] , is currently increasing [2] . The recent discovery of the efficacy of sorafenib, a multikinase inhibitor, as a treatment for patients with advanced HCC, has represented a major breakthrough in the clinical management, although the survival benefit has been shown to be less than 3 months [3] . No other effective therapy is currently available for patients with advanced disease [4] . As such, there is a continuing need to develop novel therapeutics and approaches for treatment of advanced HCC [5] . To develop targeted cancer therapies, we must first identify aberrantly regulated molecular pathways specific to this cancer. Clinically, it is also important to discover useful and convenient surrogate serum biomarkers that reflect aberrations in molecular pathways due to the molecular mechanisms of their expression, to identify the deregulated intracellular signalling pathways and to spare the patients from invasive clinical tests. Currently, α-fetoprotein (AFP) is the most widely used serum biomarker for HCC surveillance [6] . Although the regulation of AFP gene expression is not fully understood, p53 (ref. 7 ), β-catenin [8] and the recently identified zinc-finger protein, ZBTB20 (ref. 9 ), have been reported to be involved. Furthermore, whereas mounting clinical evidence indicates that AFP elevation is linked to a more aggressive tumour phenotype characterized by vascular invasion, metastasis and poor differentiation [10] , [11] , it remains to be determined whether the two phenotypes represent anything more than coincidental epiphenomena [12] . MicroRNAs (miRNAs) are short, single-stranded, non-coding RNAs. Although first identified in Caenorhabditis elegans [13] , miRNAs are now known to be expressed in most organisms, from plants to vertebrates [14] . Primary miRNAs, which possess stem-loop structures, are processed into mature miRNAs by Drosha and Dicer RNA polymerase III. These mature miRNAs then associate with the RNA-induced silencing complex, and the resulting complex directly binds to the 3′-untranslated regions of target messenger RNAs to act as suppressors of translation and gene expression. Thus, depending on the target mRNAs, miRNAs are responsible for the control of various biological functions including cell proliferation, apoptosis, differentiation, metabolism, oncogenesis and oncogenic suppression [15] , [16] , [17] . MiRNA122 (miR122) is a tissue-specific miRNA that is most abundant in the liver [18] , wherein it is responsible for the maintenance of fatty acid metabolism [19] , [20] and circadian rhythms [21] . As shown for other tissue-specific miRNAs [22] , expression of miR122 has been reported to be downregulated in carcinomas, particularly in more malignant tumours, although these results remain controversial because of conflicting reports [23] , [24] , [25] , [26] . The biological significance of the downregulation of miR122 expression in HCC at the molecular level has not yet been fully elucidated. In the present study, we explored the role of microR122 in HCC by silencing it both in human HCC cells and in a transgenic mouse model. Our molecular analysis enabled us to define the complex regulatory cascades underlying the clinically recognized link between raised AFP levels and a more aggressive phenotype in HCC. Establishment of miR122-silenced HCC cell lines To characterize the functional consequences of miR122 downregulation in HCC cells, Huh7 and PLC/PRF/5 cells were stably transduced with a lentivirus that expresses RNA hairpins that produce mature antisense RNA designed to silence miR122 function. These cells were selected on the basis of their relatively high levels of miR122 expression [24] , [27] . Several mismatches were intentionally inserted into the RNA hairpin sequences to produce more stable templates for miR122 binding and sequestration and to perturb the participation of miR122 in RNA-induced silencing complex-associated inhibition of translation ( Fig. 1a ). 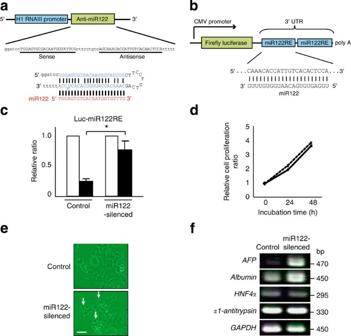Figure 1: Establishment of miR122-silenced HCC cell lines. (a), The miRZip122 construct, which yields a functional single-stranded full-length antisense miRNA complementary o miR122, processed from a stem-loop-stem molecule and transcribed from the constitutively active H1 RNA III promoter. Several mismatched nucleotides were included to efficiently produce a single-stranded antisense miR122 molecule. (b) Schematic representation of the luciferase reporter used to examine miR122 activity. The firefly luciferase gene, driven by a cytomegalovirus (CMV) promoter, contains two tandem miR122-binding sites (miR122-responsive elements; miR122-RE) in its 3′-UTR. (c) The suppressive effects of miR122 precursor expression (black bar) on luciferase activity in control and miR122-silenced cells. Test values were normalized to those obtained from the cells transfected with a miRNA precursor-non-expressing empty vector (white bar), which were set to 1. Data represent the mean±s.d. of three independent experiments using Huh7 cells. *P<0.05 (t-test). Similar results were obtained using PLC/PRF/5 cells. (d) Control (solid line) and miR122-silenced cells (dashed line) were plated at a density of 2×104cells per well. After incubation for 24 and 48 h, numbers of cells were calculated as described in the Methods. Data represent the mean±s.d. of three independent experiments using Huh7 cells. Similar results were obtained using PLC/PRF/5 cells. (e) Changes in cellular morphology of Huh7 miR122-silenced cells are shown. Arrows indicate pseudopodia. Scale bar, 50 μm. Similar phenotypes were observed using PLC/PRF/5 cells. (f) The expression of several hepatocyte markers in control and Huh7 miR122-silenced cells was evaluated by semi-quantitative RT–PCR. Representative results from three independent experiments using Huh7 cells are shown. Similar results were obtained using PLC/PRF/5 cells. Figure 1: Establishment of miR122-silenced HCC cell lines. ( a ), The miRZip122 construct, which yields a functional single-stranded full-length antisense miRNA complementary o miR122, processed from a stem-loop-stem molecule and transcribed from the constitutively active H1 RNA III promoter. Several mismatched nucleotides were included to efficiently produce a single-stranded antisense miR122 molecule. ( b ) Schematic representation of the luciferase reporter used to examine miR122 activity. The firefly luciferase gene, driven by a cytomegalovirus (CMV) promoter, contains two tandem miR122-binding sites (miR122-responsive elements; miR122-RE) in its 3′-UTR. ( c ) The suppressive effects of miR122 precursor expression (black bar) on luciferase activity in control and miR122-silenced cells. Test values were normalized to those obtained from the cells transfected with a miRNA precursor-non-expressing empty vector (white bar), which were set to 1. Data represent the mean±s.d. of three independent experiments using Huh7 cells. * P <0.05 ( t -test). Similar results were obtained using PLC/PRF/5 cells. ( d ) Control (solid line) and miR122-silenced cells (dashed line) were plated at a density of 2×10 4 cells per well. After incubation for 24 and 48 h, numbers of cells were calculated as described in the Methods. Data represent the mean±s.d. of three independent experiments using Huh7 cells. Similar results were obtained using PLC/PRF/5 cells. ( e ) Changes in cellular morphology of Huh7 miR122-silenced cells are shown. Arrows indicate pseudopodia. Scale bar, 50 μm. Similar phenotypes were observed using PLC/PRF/5 cells. ( f ) The expression of several hepatocyte markers in control and Huh7 miR122-silenced cells was evaluated by semi-quantitative RT–PCR. Representative results from three independent experiments using Huh7 cells are shown. Similar results were obtained using PLC/PRF/5 cells. Full size image To confirm effective miR122 silencing in transduced cells, we analysed the luciferase activity of reporters containing miR122-binding sites (the function of which is suppressed by miR122 overexpression) ( Fig. 1b ) in miR122-silenced and control cells. As expected, overexpression of the miR122 precursor greatly suppressed luciferase activity in control cells ( Fig. 1c ). In contrast, this suppressive effect was significantly reduced in miR122-silenced cells ( Fig. 1c ), indicating that miR122 was indeed functionally silenced. To characterize the biological changes that result from the loss of miR122 function, we next analysed cell proliferation, morphology and differentiation in miR122-silenced cells. The rates of cell proliferation were comparable between control and silenced cells ( Fig. 1d ); however, miR122-silenced cells exhibited a larger number of distinct pseudopodia ( Fig. 1e ). Next, as miR122 is specifically expressed in the liver, we hypothesized that it may have a role in hepatocyte differentiation and, therefore, we investigated the expression of several hepatocyte markers by semi-quantitative RT–PCR. We observed an increase in AFP expression and a slight elevation of albumin expression in miR122-silenced cells, but the expression levels of other hepatocyte markers, such as hepatocyte nuclear factor 4α (HNF4α) and α 1 -antitrypsin, did not change ( Fig. 1f ). MiR122-silenced HCC cells exhibit a more invasive phenotype Because miR122-silenced cells exhibited an increased number of pseudopodia, we next characterized phenotypes associated with more biologically aggressive cell characteristics. We found that actin polymerization and pseudopod formation were significantly increased in miR122-silenced cells ( Fig. 2a ). The increase in the number of pseudopodia was confirmed by a quantitative pseudopodia assay ( Supplementary Fig. S1 ). Although the expression levels of the mesenchymal marker α-smooth muscle actin were only slightly increased, we observed a significant decrease in the expression of the epithelial marker E-cadherin in miR122-silenced cells ( Fig. 2b ). Furthermore, the expression of other epithelial-to-mesenchymal transition markers such as fibronectin, N-cadherin, snail and Zeb1 was altered in miR122-silenced cells ( Supplementary Fig. S1 ). These findings are consistent with the notion that loss of miR122 function leads to a more malignant phenotype. 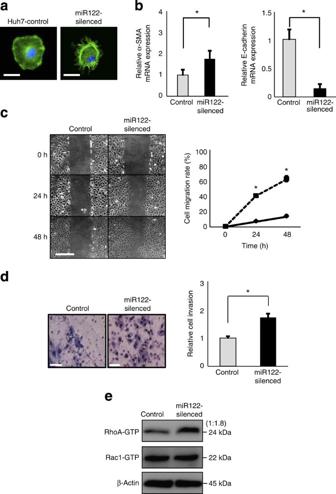Figure 2: HCC cells silenced for miR122 function exhibit a more invasive phenotype. (a) Cells were treated with 2 ng ml−1TGF-β for 12 h, and actin filaments were stained with Alexa Fluor 488-conjugated phalloidin. Representative results from two independent experiments using Huh7 cells are shown. Similar results were obtained using PLC/PRF/5 cells. Scale bar, 50 μm. (b) Expression levels of α−smooth muscle actin and E-cadherin mRNAs were assessed by quantitative RT–PCR. Values shown represent mRNA expression levels in experimental cells relative to control cells. Data represent the mean±s.d. of three independent experiments using Huh7 cells. *P<0.05 (t-test). Similar results were obtained for PLC/PRF/5 cells. (c) The degree of cell migration was characterized using a scratch assay. The ratio of migrating cells was significantly increased in miR122-silenced cells at 24 and 48 h after scratching. Left panels show representative images. Right panel shows the results from cell counts for four randomly chosen fields per experiment. Data are represented as the mean±s.d. of three experiments using Huh7 control (solid line) and miR122-silenced cells (dashed line). *P<0.001 (t-test). Similar results were obtained for PLC/PRF/5 cells. (d) The degree of cell invasion was examined using cell invasion chambers. Representative images of stained invaded cells (left). The relative cell invasion ratio after normalization to control cell invasion levels (right). Data represent the mean±s.d. of three independent experiments using Huh7 cells. Scale bar, 100 μm. *P<0.01 (t-test). Similar results were obtained for PLC/PRF/5 cells. (e) Rho and Rac1 activity was determined by comparing the amounts of active GTP-bound RhoA (RhoA-GTP) and Rac1 (Rac1-GTP) between control and miR122-silenced cells. The indicated numbers represent the relative expression levels. Equal loading in pull-down assays was confirmed by analysis of β-actin levels in the cell lysates. Representative results of five independent experiments using Huh7 cells are shown. Similar results were obtained using PLC/PRF/5 cells. Figure 2: HCC cells silenced for miR122 function exhibit a more invasive phenotype. ( a ) Cells were treated with 2 ng ml −1 TGF-β for 12 h, and actin filaments were stained with Alexa Fluor 488-conjugated phalloidin. Representative results from two independent experiments using Huh7 cells are shown. Similar results were obtained using PLC/PRF/5 cells. Scale bar, 50 μm. ( b ) Expression levels of α−smooth muscle actin and E-cadherin mRNAs were assessed by quantitative RT–PCR. Values shown represent mRNA expression levels in experimental cells relative to control cells. Data represent the mean±s.d. of three independent experiments using Huh7 cells. * P <0.05 ( t -test). Similar results were obtained for PLC/PRF/5 cells. ( c ) The degree of cell migration was characterized using a scratch assay. The ratio of migrating cells was significantly increased in miR122-silenced cells at 24 and 48 h after scratching. Left panels show representative images. Right panel shows the results from cell counts for four randomly chosen fields per experiment. Data are represented as the mean±s.d. of three experiments using Huh7 control (solid line) and miR122-silenced cells (dashed line). * P <0.001 ( t -test). Similar results were obtained for PLC/PRF/5 cells. ( d ) The degree of cell invasion was examined using cell invasion chambers. Representative images of stained invaded cells (left). The relative cell invasion ratio after normalization to control cell invasion levels (right). Data represent the mean±s.d. of three independent experiments using Huh7 cells. Scale bar, 100 μm. * P <0.01 ( t -test). Similar results were obtained for PLC/PRF/5 cells. ( e ) Rho and Rac1 activity was determined by comparing the amounts of active GTP-bound RhoA (RhoA-GTP) and Rac1 (Rac1-GTP) between control and miR122-silenced cells. The indicated numbers represent the relative expression levels. Equal loading in pull-down assays was confirmed by analysis of β-actin levels in the cell lysates. Representative results of five independent experiments using Huh7 cells are shown. Similar results were obtained using PLC/PRF/5 cells. Full size image We next performed scratch and invasion assays to characterize the invasive phenotype of miR122-silenced cells. Rates of cell migration and of cell invasion were significantly increased in miR122-silenced cells ( Fig. 2c,d ). As the proliferation rates of control and miR122-silenced cells were similar ( Fig. 1d ), altogether these results suggest that inhibition of miR122 function in HCC cells may lead to increases in malignancy-related cellular properties. To investigate the molecular mechanisms underlying these cellular phenotypes, we assessed the activity of RhoA and Rac1,which are small GTPases that are closely associated with cell migration and invasion [28] . Although Rac1 activity did not significantly change, RhoA activity significantly increased in miR122-silenced cells ( Fig. 2e ), suggesting that the increase in cell migration and invasion in miR122-silenced cells may result from increased RhoA activity. AFP expression is increased in miR122-silenced HCC cells As we observed an increase in AFP expression in miR122-silenced cells ( Fig. 1f ), we next sought to quantify AFP concentrations in culture supernatants using an enzyme-linked immunosorbent assay (ELISA). AFP levels were approximately three times higher in the supernatant of miR122-silenced cells as compared with control cells ( Fig. 3a ). Consistent with this observation, immunofluorescence staining for AFP produced a stronger cytoplasmic signal and quantitative RT–PCR revealed a tenfold increase in AFP mRNA levels in miR122-silenced cells ( Fig. 3b,c ). 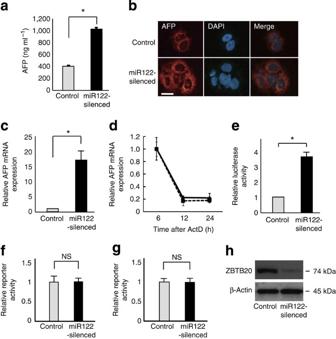Figure 3: Increased expression of AFP in HCC cells silenced for miR122 function. (a) The AFP concentration in the culture medium was determined by ELISA. Data represent the mean±s.d. of three independent experiments using Huh7 cells. *P<0.01 (t-test). Similar results were obtained for PLC/PRF/5 cells. (b) Immunofluorescent staining for AFP in the cytoplasm of control and miR122-silenced Huh7cells. Representative images of stained cells from three independent experiments are shown. Scale bar, 50 μm. (c) Amounts of AFP mRNA in Huh7 control and miR122-silenced cells were determined by quantitative RT–PCR. Data represent the mean±s.d. of three independent experiments. *P<0.05 (t-test). Similar results were obtained using PLC/PRF/5 cells. (d) AFP mRNA stability in Huh7 control (solid line) and miR122-silenced (dashed line) cells was determined by quantitative RT–PCR at 6, 12, and 24 h after treating cells with 10 μl ml−1actinomycin D. Data represent the mean±s.d. of three independent experiments. Similar results were observed using PLC/PRF/5 cells. (e) AFP promoter activity was measured in reporter assays using Huh7 cells and AFP promoter-luciferase construct. Data represent the mean±s.d. of three independent experiments. *P<0.05 (t-test). Similar results were obtained using PLC/PRF/5 cells. (f,g) Luciferase assays were performed using reporter plasmids to measure p53 (f) and β-catenin (g) activities. Data represent the mean±s.d. of three independent experiments. Similar results were obtained using PLC/PRF/5 cells. (h) ZBTB20 protein levels in miR122-silenced cells. A representative result from three independent experiments using Huh7 cells is shown. Similar results were obtained using PLC/PRF/5 cells. Figure 3: Increased expression of AFP in HCC cells silenced for miR122 function. ( a ) The AFP concentration in the culture medium was determined by ELISA. Data represent the mean±s.d. of three independent experiments using Huh7 cells. * P <0.01 ( t -test). Similar results were obtained for PLC/PRF/5 cells. ( b ) Immunofluorescent staining for AFP in the cytoplasm of control and miR122-silenced Huh7cells. Representative images of stained cells from three independent experiments are shown. Scale bar, 50 μm. ( c ) Amounts of AFP mRNA in Huh7 control and miR122-silenced cells were determined by quantitative RT–PCR. Data represent the mean±s.d. of three independent experiments. * P <0.05 ( t -test). Similar results were obtained using PLC/PRF/5 cells. ( d ) AFP mRNA stability in Huh7 control (solid line) and miR122-silenced (dashed line) cells was determined by quantitative RT–PCR at 6, 12, and 24 h after treating cells with 10 μl ml −1 actinomycin D. Data represent the mean±s.d. of three independent experiments. Similar results were observed using PLC/PRF/5 cells. ( e ) AFP promoter activity was measured in reporter assays using Huh7 cells and AFP promoter-luciferase construct. Data represent the mean±s.d. of three independent experiments. * P <0.05 ( t -test). Similar results were obtained using PLC/PRF/5 cells. ( f , g ) Luciferase assays were performed using reporter plasmids to measure p53 ( f ) and β-catenin ( g ) activities. Data represent the mean±s.d. of three independent experiments. Similar results were obtained using PLC/PRF/5 cells. ( h ) ZBTB20 protein levels in miR122-silenced cells. A representative result from three independent experiments using Huh7 cells is shown. Similar results were obtained using PLC/PRF/5 cells. Full size image The 3′-UTR of the AFP mRNA did not contain predicted miR122 target sequences, based on sequence analyses performed using miRNA target search engines such as TargetScan ( http://www.targetscan.org ), suggesting that it is unlikely that miR122 directly regulates AFP expression. Therefore, to characterize the mechanisms underlying increased AFP expression in miR122-silenced cells, we first assessed the stability of the AFP mRNA in miR122-silenced cells. As expected, AFP mRNA stability was unaffected by silencing of miR122, as the amount of mRNA was comparable between control and miR122-silenced cells at 6, 12 and 24 h after inhibition of new transcription by treatment with actinomycin D ( Fig. 3d ). The increase in AFP mRNA levels in the absence of changes in mRNA stability suggested that transcription of AFP was increased in miR122-silenced cells as a result of increased AFP promoter activity. Indeed, AFP promoter activity was almost four times higher in miR122-silenced cells than in control cells, as assessed by a reporter assay ( Fig. 3e ). Because AFP promoter activity is in part regulated by p53 (ref. 7 ), we assessed p53 activity using reporter constructs. However, no changes in p53 activity were detected in miR122-silenced cells ( Fig. 3f ). As mutation of β-catenin has also been reported to be involved in upregulation of AFP expression [8] , we next analysed β-catenin activity in miR122-silenced cells. Similar to p53, no change in β-catenin activity was evident in miR122-silenced cells compared with control cells ( Fig. 3g ). Recently, it was reported that ZBTB20 acts as a repressor of AFP transcription [9] . This result led us to assess the expression of the ZBTB20 protein in miR122-silenced cells. Indeed, western blot analysis revealed that ZBTB20 expression was decreased in miR122-silenced cells ( Fig. 3h ). However, as ZBT20 lacks the presence of predicted miR122 target sequences based on computational searches of the 3′-UTR, it was also unlikely that miR122 directly regulates ZBTB20 expression. These observations suggest that other indirect mechanisms may lead to decreased ZBTB20 expression in miR122-silenced cells. CUX1 is the regulator of phenotypes in miR122-silenced cells To explore the mechanisms by which miR122 regulates cell motility, invasion and AFP expression, we used computational searches to identify potential miR122 target genes with known functions related to these processes. This analysis led to the identification of Cut homeobox 1 (CUX1, also known as CCAAT-displacement protein/cut homeobox, CDP/Cux/Cut) through the presence of a high probability miR122 target site located in the 3′-UTR and a perfect match in the seed sequences. CUX1 is a transcription factor that regulates multiple processes including cell cycle progression, chromosomal segregation and cell migration [29] , [30] . Consistent with the effects of miR122 silencing described above, CUX1 was reported to modulate cell motility and invasion through the control of RhoA activity [31] , [32] , [33] . We observed that whereas CUX1 mRNA levels remained unchanged ( Fig. 4a ), there was a significant increase in the steady-state level of the CUX1 p200 and p110 isoforms in miR122-silenced cells ( Fig. 4b ). 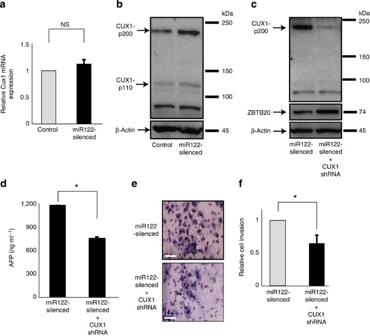Figure 4: CUX1-mediated regulation of AFP expression and phenotypic changes in miR122 functionally silenced cells. (a) CUX1 mRNA levels in control and miR122-silenced cells were analysed by quantitative RT–PCR. Data represent the mean±s.d. of three independent experiments using Huh7 cells. (b) p200 and p110 CUX1 protein levels were increased in miR122-silenced cells compared with control cells. A representative result from three independent experiments using Huh7 cells is shown. Similar results were obtained for PLC/PRF/5 cells. (c) CUX1 and ZBTB20 protein expression in double CUX1/miR122 knockdown Huh7 cells. Similar results were obtained using PLC/PRF/5 cells. (d) AFP concentrations in the culture medium supernatants were determined by ELISA. Data represent the mean±s.d. of three independent experiments. *P<0.01 (t-test). Similar results were observed using PLC/PRF/5 cells. (e,f) The change of cell invasion ratio by CUX1 knockdown in miR122-silenced Huh7 cells. Representative images of stained invading cells are shown (e). The relative cell invasion ratio after normalization to control invasion levels is shown (f). Data represent the mean±s.d. of three independent experiments. Scale bar, 100 μm. *P<0.01 (t-test). Similar results were obtained using PLC/PRF/5 cells. Figure 4: CUX1-mediated regulation of AFP expression and phenotypic changes in miR122 functionally silenced cells. ( a ) CUX1 mRNA levels in control and miR122-silenced cells were analysed by quantitative RT–PCR. Data represent the mean±s.d. of three independent experiments using Huh7 cells. ( b ) p200 and p110 CUX1 protein levels were increased in miR122-silenced cells compared with control cells. A representative result from three independent experiments using Huh7 cells is shown. Similar results were obtained for PLC/PRF/5 cells. ( c ) CUX1 and ZBTB20 protein expression in double CUX1/miR122 knockdown Huh7 cells. Similar results were obtained using PLC/PRF/5 cells. ( d ) AFP concentrations in the culture medium supernatants were determined by ELISA. Data represent the mean±s.d. of three independent experiments. * P <0.01 ( t -test). Similar results were observed using PLC/PRF/5 cells. ( e , f ) The change of cell invasion ratio by CUX1 knockdown in miR122-silenced Huh7 cells. Representative images of stained invading cells are shown ( e ). The relative cell invasion ratio after normalization to control invasion levels is shown ( f ). Data represent the mean±s.d. of three independent experiments. Scale bar, 100 μm. * P <0.01 ( t -test). Similar results were obtained using PLC/PRF/5 cells. Full size image To investigate the contribution of CUX1 upregulation to the increase in AFP expression and invasive properties observed in miR122-silenced cells, we knocked down CUX1 protein expression using lentiviruses expressing CUX1 short hairpin RNAs (shRNAs) ( Fig. 4c ). In the resulting double-knockdown cells, AFP protein expression in cell-culture supernatant and cell invasion were both reduced to levels similar to that of the parental Huh7 cells ( Fig. 4d–f ). CUX1 represses ZBTB20 expression via miR214 We next assessed whether miR122 directly targets CUX1 by constructing a luciferase reporter construct that possessed a portion of the CUX1 3′-UTR containing the putative miR122 target site ( Fig. 5a ). Co-transfection experiments revealed that luciferase activity was suppressed by overexpression of a miR122 precursor-expressing plasmid ( Fig. 5b ). This suppressive effect was prevented by introducing two point mutations into the seed sequences of the miR122 target site ( Fig. 5a,b ), demonstrating that miR122 directly targets these sequences. 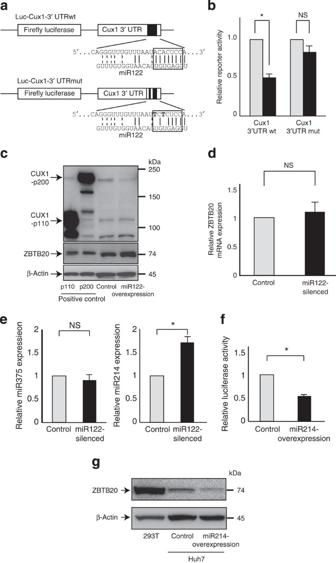Figure 5: MiR122 directly targets CUX1. (a) A luciferase reporter carrying a region of the wild type CUX1 3′UTR containing the putative miR122 target site (Luc-CUX1-3′UTRwt) was used to assess the effects of miR122 on expression of CUX1. A second luciferase reporter with two nucleotide mutations (indicated in bold) in the seed sequences (indicated by a rectangle) of the putative miR122 target sites (Luc-CUX1-3′UTRmut) was also utilized to assess specificity. (b) Huh7 cells were co-transfected with Luc-CUX1-3′UTRwt or Luc-CUX1-3′UTRmut and either an empty control vector (white bar) or a miR122 precursor expression plasmid (black bar). Data represent the mean±s.d. of three independent experiments. *P<0.05 (t-test). (c) CUX1 and ZBTB20 expression in 293 T cells-expressing the miR122 precursor. Cell lysates transiently transfected with CUX1 p200 or p110 expression plasmids were used as positive controls. Representative results from four independent experiments are shown. (d) ZBTB20 mRNA levels in miR122-silenced Huh7 cells were determined by quantitative RT–PCR. Data represent the mean±s.d. of three independent experiments. Similar results were obtained using PLC/PRF/5 cells. (e) Levels of miR375 (left) and miR214 (right) in miR122-silenced Huh7 cells were analysed by quantitative RT–PCR. Data represent the mean±s.d. of three independent experiments. *P<0.05 (t-test). (f) Huh7 cells were co-transfected with Luc-ZBTB20-3′UTR and either an empty control vector or an miR214 precursor expression plasmid. Data represent the mean±s.d. of three independent experiments. *P<0.05 (t-test). (g) ZBTB20 expression was decreased in Huh7 miR214-overexpressing cells. 293T cell lysate was used as a positive control. Representative results from four independent experiments are shown. Figure 5: MiR122 directly targets CUX1. ( a ) A luciferase reporter carrying a region of the wild type CUX1 3′UTR containing the putative miR122 target site (Luc-CUX1-3′UTRwt) was used to assess the effects of miR122 on expression of CUX1. A second luciferase reporter with two nucleotide mutations (indicated in bold) in the seed sequences (indicated by a rectangle) of the putative miR122 target sites (Luc-CUX1-3′UTRmut) was also utilized to assess specificity. ( b ) Huh7 cells were co-transfected with Luc-CUX1-3′UTRwt or Luc-CUX1-3′UTRmut and either an empty control vector (white bar) or a miR122 precursor expression plasmid (black bar). Data represent the mean±s.d. of three independent experiments. * P <0.05 ( t -test). ( c ) CUX1 and ZBTB20 expression in 293 T cells-expressing the miR122 precursor. Cell lysates transiently transfected with CUX1 p200 or p110 expression plasmids were used as positive controls. Representative results from four independent experiments are shown. ( d ) ZBTB20 mRNA levels in miR122-silenced Huh7 cells were determined by quantitative RT–PCR. Data represent the mean±s.d. of three independent experiments. Similar results were obtained using PLC/PRF/5 cells. ( e ) Levels of miR375 (left) and miR214 (right) in miR122-silenced Huh7 cells were analysed by quantitative RT–PCR. Data represent the mean±s.d. of three independent experiments. * P <0.05 ( t -test). ( f ) Huh7 cells were co-transfected with Luc-ZBTB20-3′UTR and either an empty control vector or an miR214 precursor expression plasmid. Data represent the mean±s.d. of three independent experiments. * P <0.05 ( t -test). ( g ) ZBTB20 expression was decreased in Huh7 miR214-overexpressing cells. 293T cell lysate was used as a positive control. Representative results from four independent experiments are shown. Full size image To confirm these effects, we generated 293T cell lines that stably expressed the miR122-precursor construct by transducing cells with miR122 precursor-expressing lentiviruses tagged with green fluorescent protein ( Supplementary Fig. S2a ). As expected, the anti-miR122 construct did not affect control 293T cells, owing to the lack of miR122 expression. However, the anti-miR122 construct greatly enhanced luciferase activity in 293T cells stably expressing the miR122-precursor, confirming that miR122 was transduced into the 293 T cells ( Supplementary Fig. S2b ). Consistent with the results described above, these cells exhibited decreased expression of CUX1, particularly the p200 isoform, and also showed a modest, but reproducible, increase in ZBTB20 expression ( Fig. 5c ). These results suggest that miR122 directly regulates CUX1 protein expression, which in turn may regulate ZBTB20 expression. Because CUX1 can function as a transcriptional modulator [29] , we initially hypothesized that CUX1 is a direct regulator of ZBTB20 transcription. However, quantitative RT–PCR analysis revealed that levels of the ZBTB20 mRNA were unchanged in miR122-silenced cells compared with controls ( Fig. 5d ). To explain the discrepancy between unchanged levels of ZBTB20 mRNA and decreases in protein expression levels in miR122-silenced cells, we searched for miRNAs that could potentially target the ZBTB20 3′-UTR. Based on computational searches, miR214 and miR375 were identified as candidate ZBTB20-regulatory miRNAs. Although levels of miR375 were unchanged in miR122-silenced cells ( Fig. 5e ), expression of miR214 was significantly increased ( Fig. 5e ). To assess whether miR214 directly targeted the ZBTB20 3′-UTR, we constructed a luciferase reporter with the region of the ZBTB20 3′-UTR that contains the putative miR214 target site. Reporter assays revealed that luciferase activity was indeed suppressed by overexpression of the miR214 precursor, suggesting that miR214 directly targets the ZBTB20 3′-UTR and suppresses its expression ( Fig. 5f ). Consistent with these findings, cells that stably overexpressed the miR214 precursor exhibited decreased levels of ZBTB20 protein expression ( Fig. 5g ). The putative promoter regions of miR214 contain multiple CUX1 binding sites as revealed by MATCH, a transcription factor binding site search engine ( http://www.gene-regulation.com ). A scanning chromatin immunoprecipitation (ChIP) experiment, followed by real-time PCR, using a series of primer pairs, confirmed that CUX1 binds to multiple genomic sites in the miR214 promoter region ( Fig. 6a ). We therefore hypothesized that CUX1 may regulate miR214 transcription. Consistent with this notion, we found that miR214 expression was decreased in CUX1 knockdown Huh7 cells ( Fig. 6b ). The role of CUX1 as an activator of miR214 transcription was further verified by knocking down or overexpressing CUX1 in another cell line. Levels of miR214 decreased following the constitutive knockdown of CUX1 with shRNA ( Fig. 6c ). In contrast, retroviral infection with a vector expressing p110 CUX1 led to an increase in miR214 ( Fig. 6d ). These findings were confirmed using doxycycline-inducible CUX1 shRNA. As previously observed for other transcriptional targets of CUX1 (refs 30 , 34 ), levels of miR214 were reduced in the presence of doxycycline, and then returned to levels higher than in untreated cells upon removal of the doxycycline inducer miR214 ( Fig. 6e ). 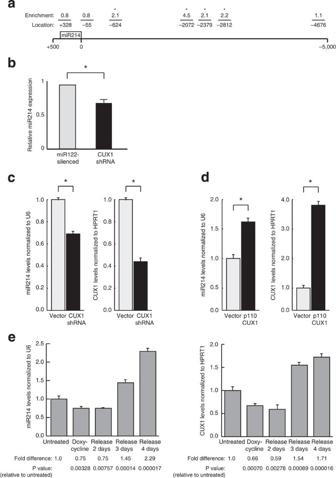Figure 6: CUX1 regulated miR-214 expression. (a), CUX1 enrichment at the miR214 locus. ChIP assays were performed using Hs578T cells. Fold enrichment and location of the center of each qPCR amplicon are shown. *P<0.05 (t-test). (b) MiR214 expression levels after CUX1 knockdown in miR122-silenced Huh7 cells were determined by quantitative RT–PCR. Data represent the mean±s.d. of three independent experiments. *P<0.05 (t-test). Similar results were obtained using PLC/PRF/5 cells. (c) Levels of miR214 and CUX1 RNA in Hs578T cells infected with an empty vector or a lentiviral vector constitutively expressing CUX1 shRNA. Data represent the mean±s.d. of three independent experiments. *P<0.05 (t-test). (d) Hs578T cells were infected with a retrovirus expressing p110 CUX1. Levels of miR214 and CUX1 mRNA were measured 1 day later. Data represent the mean±s.d. of three independent experiments. *P<0.05 (t-test). (e) Levels of miR214 and CUX1 mRNA in Hs578T cells expressing a doxycycline-inducible CUX1 shRNA. Levels are shown prior to treatment, after 5 days of doxycycline treatment, and 2, 3 and 4 days after withdrawal of doxycycline. Fold changes with the mean±s.d. of three independent experiments andP-values are shown (t-test). Figure 6: CUX1 regulated miR-214 expression. ( a ), CUX1 enrichment at the miR214 locus. ChIP assays were performed using Hs578T cells. Fold enrichment and location of the center of each qPCR amplicon are shown. * P <0.05 ( t -test). ( b ) MiR214 expression levels after CUX1 knockdown in miR122-silenced Huh7 cells were determined by quantitative RT–PCR. Data represent the mean±s.d. of three independent experiments. * P <0.05 ( t -test). Similar results were obtained using PLC/PRF/5 cells. ( c ) Levels of miR214 and CUX1 RNA in Hs578T cells infected with an empty vector or a lentiviral vector constitutively expressing CUX1 shRNA. Data represent the mean±s.d. of three independent experiments. * P <0.05 ( t -test). ( d ) Hs578T cells were infected with a retrovirus expressing p110 CUX1. Levels of miR214 and CUX1 mRNA were measured 1 day later. Data represent the mean±s.d. of three independent experiments. * P <0.05 ( t -test). ( e ) Levels of miR214 and CUX1 mRNA in Hs578T cells expressing a doxycycline-inducible CUX1 shRNA. Levels are shown prior to treatment, after 5 days of doxycycline treatment, and 2, 3 and 4 days after withdrawal of doxycycline. Fold changes with the mean±s.d. of three independent experiments and P -values are shown ( t -test). Full size image Next, to assess the contribution of miR214 to the control of ZBTB20 expression in miR122-silenced cells, we measured ZBTB20 expression after parallel silencing of miR214 in miR122-silenced cells. Although ZBTB20 protein expression was reduced by almost 50% by miR122 silencing, it was restored to >90% of control levels by miR214 silencing ( Supplementary Fig. S3 ). Thus, CUX1-induced miR214 regulates, at least in part, ZBTB20 expression in miR122-silenced cells, leading to the upregulation of AFP expression. Regulation of of CUX1 and AFP expression by miR122 was also confirmed in other HCC cell lines in which miR122 was overexpressed or silenced. Northern blotting showed that the expression of miR122 was relatively low in Hep3B and HepG2 cells, but was relatively high in Huh1, Huh7 and PLC/PRF/5 cells ( Supplementary Fig. S4a ). We therefore overexpressed the miR122 precursor in Hep3B and HepG2 cells and silenced miR122 in Huh1, Huh7 and PLC/PRF/5 cells ( Supplementary Fig. S4b ). CUX1 expression was respectively suppressed and enhanced by miR122 precursor overexpression and miR122 silencing ( Supplementary Fig. S4c ). In contrast, AFP expression was respectively enhanced and suppressed ( Supplementary Fig. S4d ), confirming that AFP expression is regulated by an miR122-CUX1 pathway in multiple HCC cell lines. These results indicate that functional silencing of miR122 leads to an increase in CUX1 protein expression, resulting in repression of ZBTB20 through an increase in miR214 expression. Repression of ZBTB20, in turn, leads to an increase in AFP expression. Because CUX1 is a modulator of cell motility and invasion [35] , [36] , [37] , upregulation of this protein also enhances RhoA activity, increasing the malignant properties of cancer cells. Expression of CUX1-related molecules in miR122-silenced mice To explore the pathway delineated above in an in vivo model, we generated transgenic mice expressing antisense miR122 under the control of an H1 promoter ( Fig. 7a ) to inhibit the function of endogenous miR122 (ref. 38 ). In situ hybridization analysis in these mice revealed weak miR122 staining in liver tissue in comparison with control mice, likely due to binding of the anti-sense miR122 to endogenous miR122, which produces a double-stranded DNA and likely inhibits hybridization of the probe ( Fig. 7b ). Although structural development of the liver appeared normal based on haematoxylin and eosin staining ( Supplementary Fig. S5 ), AFP mRNA expression ( Fig. 7c ) and p200 and p110 CUX1 protein expression were upregulated in the liver of anti-miR122 transgenic mice ( Fig. 7d ). Moreover, whereas levels of ZBTB20 mRNA were unchanged, ZBTB20 protein expression was decreased in the liver ( Fig. 7d ), in agreement with in vitro results demonstrating the regulation of ZBTB20 at the translational level ( Fig. 5c,d ). This was associated with a significant increase in the levels of miR214 in anti-miR122 transgenic mice ( Fig. 7e ). Thus, results from mouse liver tissue confirm that the miR122/CUX1/miR214/ZBTB20 regulatory pathway is also functional in an in vivo model. 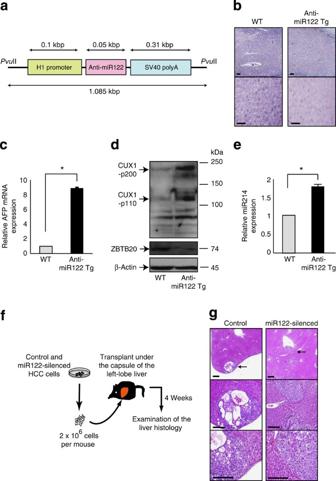Figure 7: AFP expression is increased in the liver of anti-miR122 transgenic mice. (a) DNA construct used to establishment transgenic mice in which miR122 is functionally silenced (anti-miR122 transgenic mice). This construct (like the construct used in thein vitrostudies) generates a functional single-stranded full-length antisense miRNA complementary to miR122. (b) Confirmation of the expression of an antisense RNA directed against miR122 in anti-miR122 transgenic (anti-miR122 Tg) mice. Amounts of miR122 detected byin situhybridization (blue/purple staining) in the liver tissues of anti-miR122 transgenic mice and WT mice. Results shown are representative of three independent experiments performed using littermates from four different mouse lines. Scale bar, 100 μm. No specific staining was observed when a negative control probe (LNA-scramble) was used. (c) AFP mRNA expression in mouse liver tissues was analysed by quantitative RT–PCR. Data represent the mean±s.d. of results for five mice in each group. *P<0.05 (t-test). (d) CUX1 and ZBTB20 expression in mouse liver tissues was assessed by Western blotting. A representative result from three independent experiments is shown. (e) Levels of miR214 in liver tissues were determined by quantitative RT–PCR. Data represent the mean±s.d. of three independent experiments. *P<0.05 (t-test). (f) Protocols of the orthotopic xenograft models of HCC cells. Control and miR122-silenced PLC/PRF/5 cells were prepared and injected under the capsule of the left-lobe of the nude mouse liver. Six mice were included in each group. At 4 weeks after transplantation, liver tissues were collected and sliced in series. Histological examination by H&E staining was performed to examine the tumour cell invasion status. (g) Representative liver histology images at 4 weeks after transplantation of tumour cells are shown. Whereas only the transplanted HCC cells beneath the capsule of the liver edge could be detected (arrow, upper left panel), neither intrahepatic metastasis nor vascular invasion was observed in the livers of mice transplanted with control cells. In contrast, vascular invasion by multiple tumour cells (arrow, upper right panel) was observed in mice transplanted with miR122-silenced cells. Scale bar, 500 μm. WT, wild type. Figure 7: AFP expression is increased in the liver of anti-miR122 transgenic mice. ( a ) DNA construct used to establishment transgenic mice in which miR122 is functionally silenced (anti-miR122 transgenic mice). This construct (like the construct used in the in vitro studies) generates a functional single-stranded full-length antisense miRNA complementary to miR122. ( b ) Confirmation of the expression of an antisense RNA directed against miR122 in anti-miR122 transgenic (anti-miR122 Tg) mice. Amounts of miR122 detected by in situ hybridization (blue/purple staining) in the liver tissues of anti-miR122 transgenic mice and WT mice. Results shown are representative of three independent experiments performed using littermates from four different mouse lines. Scale bar, 100 μm. No specific staining was observed when a negative control probe (LNA-scramble) was used. ( c ) AFP mRNA expression in mouse liver tissues was analysed by quantitative RT–PCR. Data represent the mean±s.d. of results for five mice in each group. * P <0.05 ( t -test). ( d ) CUX1 and ZBTB20 expression in mouse liver tissues was assessed by Western blotting. A representative result from three independent experiments is shown. ( e ) Levels of miR214 in liver tissues were determined by quantitative RT–PCR. Data represent the mean±s.d. of three independent experiments. * P <0.05 ( t -test). ( f ) Protocols of the orthotopic xenograft models of HCC cells. Control and miR122-silenced PLC/PRF/5 cells were prepared and injected under the capsule of the left-lobe of the nude mouse liver. Six mice were included in each group. At 4 weeks after transplantation, liver tissues were collected and sliced in series. Histological examination by H&E staining was performed to examine the tumour cell invasion status. ( g ) Representative liver histology images at 4 weeks after transplantation of tumour cells are shown. Whereas only the transplanted HCC cells beneath the capsule of the liver edge could be detected (arrow, upper left panel), neither intrahepatic metastasis nor vascular invasion was observed in the livers of mice transplanted with control cells. In contrast, vascular invasion by multiple tumour cells (arrow, upper right panel) was observed in mice transplanted with miR122-silenced cells. Scale bar, 500 μm. WT, wild type. Full size image Invasiveness of miR122-silenced cells in xenograft model Next, we transplanted control and miR122-silenced PLC/PRF/5 cells under the liver capsule of nude mice ( Fig. 7f ) to determine whether miR122 silencing in HCC actually produces a more malignant phenotype in vivo . PLC/PRF/5 cells were chosen because of their transplantability in nude mice [39] . Neither intrahepatic metastases nor vascular invasion were detected in the livers of mice transplanted with control cells at 4 weeks post-transplantation. In contrast, vascular invasion was observed in the livers of mice transplanted with miR122-silenced HCC cells ( Fig. 7g ). These results suggest that miR122 silencing in HCC leads to a more aggressive phenotype. HCC staging and the expression of miR122-related molecules To assess the relevance of these results to human disease, we examined miR122 and AFP expression in several clinical-grade human HCC samples. We analysed miR122 expression by in situ hybridization ( Fig. 8a ) and AFP expression by immunohistochemistry ( Fig. 8b ). Both AFP expression and malignancy grading were inversely correlated with miR122 expression levels ( Fig. 8c,d ). In addition, CUX1, miR214 and ZBTB20 expression was also correlated with miR122 expression, as determined using serial sections ( Supplementary Fig. S6a, b and c ). These results, together with our studies in tissue culture systems and a transgenic mouse model, suggest that a reduction in the expression of miR122 increases AFP expression via a miRNA122-CUX1-miRNA214-ZBTB20 pathway and that the development of more biologically aggressive forms of HCC occurs via a miRNA122-CUX1-RhoA pathway ( Supplementary Fig. S7 ). The miRNA-mediated mechanism described in this report may explain the clinically known link between increased AFP levels and more biologically aggressive cell characteristics in HCC. 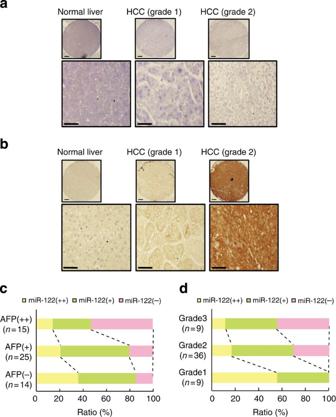Figure 8: AFP expression and HCC grade are inversely correlated with miR122 expression in human HCC samples. (a)Expression of miR122 in human clinical samples was assessed byin situhybridization. Expression of miR122 (blue/purple staining) in grade 2 (more malignant) HCC samples was less than that of normal human liver tissues or grade 1 (less malignant) HCC samples. Representative images are shown. Nuclei were stained with FastRed. Scale bar, 500 μm. (b) AFP expression, shown in brown, was analysed by immunohistochemistry. AFP expression was higher in grade 2 HCC samples than in normal human liver tissue or grade 1 HCC samples in most cases. Representative images are shown. Scale bar, 500 μm. (c) Graph shows the correlation between miR122 and AFP expression. Increased AFP expression was correlated with decreased miR122 expression. (d) Graph shows the correlation between miR122 expression and malignancy grading of HCC. Increases in malignancy grading were correlated with decreases in miR122 expression. Figure 8: AFP expression and HCC grade are inversely correlated with miR122 expression in human HCC samples. ( a) Expression of miR122 in human clinical samples was assessed by in situ hybridization. Expression of miR122 (blue/purple staining) in grade 2 (more malignant) HCC samples was less than that of normal human liver tissues or grade 1 (less malignant) HCC samples. Representative images are shown. Nuclei were stained with FastRed. Scale bar, 500 μm. ( b ) AFP expression, shown in brown, was analysed by immunohistochemistry. AFP expression was higher in grade 2 HCC samples than in normal human liver tissue or grade 1 HCC samples in most cases. Representative images are shown. Scale bar, 500 μm. ( c ) Graph shows the correlation between miR122 and AFP expression. Increased AFP expression was correlated with decreased miR122 expression. ( d ) Graph shows the correlation between miR122 expression and malignancy grading of HCC. Increases in malignancy grading were correlated with decreases in miR122 expression. Full size image High AFP levels have been clinically shown to be an unfavourable prognostic factor in HCC patients [40] . In this study, we demonstrate that reduced expression of miR122 in HCC cells contributes to elevated AFP expression and, subsequently, a more aggressive phenotype. These results provide a molecular framework that explains the reported link between elevated AFP levels and a poor clinical outcome in HCC patients. Clinically, high AFP expression is correlated with more biologically aggressive properties of HCC, as patients with high AFP levels have a significantly higher frequency of portal vein invasion and intrahepatic metastases. Additionally, these patients display significantly lower rates of recurrence-free survival and a trend towards lower overall survival [41] . In the present study, we have presented several lines of evidence indicating that decreased expression of miR122 in HCC leads to the two phenomena that are frequently observed simultaneously in the clinic: elevated expression of AFP and a more malignant biological phenotype. First, elevated AFP expression and greater cellular invasiveness were observed in miR122-knockdown cells in vitro and in vivo . Second, CUX1, which is linked with invasive characteristics in carcinoma cells [32] , [36] , [37] , was shown to be involved in regulation of AFP expression and was identified as a direct target of miR122. Third, in human tissue samples from HCC patients, inverse correlations were observed between miR122 expression and AFP expression, and between miR122 expression and tumour grade. These data suggest that it is unlikely that the clinical correlation between elevated AFP levels and a more biologically aggressive phenotype in HCC is a coincidental epiphenomenon, but, instead provide a possible molecular explanation for the decrease in miR122 expression in HCC cells. A recent study on liver development reported that liver-enriched transcription factors activate the expression of miR122, which in turn was found to promote terminal differentiation of hepatocytes through the silencing of CUX1 (ref. 42 ). In the present study, we confirmed that CUX1 is a direct target of miR122 and, in contrast to the situation in normal development, we showed that in grade 2 HCCs the decrease in miR122 is associated with higher CUX1 expression. High CUX1 expression was previously shown to inversely correlate with relapse-free and overall survival in high-grade breast cancers [36] . In transgenic mice, CUX1 was reported to cause various cancer-associated disorders depending on the specific isoform and tissue type expression [34] , [43] , [44] , [45] , [46] . In particular, expression of CUX1 caused organomegaly in several organs including the liver [43] . Hepatomegaly was associated with progression of lesions beginning with inflammation and leading to the development of mixed cell foci, hyperplasia and even HCCs, although in this last case statistical significance was not achieved because of the small size of the transgenic cohort [47] . The underlying mechanisms for the role of CUX1 in cancer is complex and is likely to involve both cell-autonomous and non-cell autonomous effects. However, from cell-based assays it is clear that CUX1 has a role in at least three distinct processes: cell motility, cell cycle progression and chromosome segregation [30] , [31] , [36] , [48] . The knockdown of CUX1 using siRNA was shown to delay entry into S phase and to hinder cell motility and invasion [31] , [36] , [48] . In contrast, overexpression of p110 CUX1 was able to accelerate S phase entry and to stimulate proliferation, migration and invasion [35] , [48] . Moreover, CUX1 was shown to promote genomic instability following cytokinesis failure [30] Regulation of AFP gene expression is a complex process mediated by a number of transcriptional activators and repressors that bind the AFP gene [7] , [8] . ZBTB20 was recently identified as a potent repressor of AFP transcription in knockout mouse studies [9] . Our results demonstrate that decreased miR122 expression leads to concomitant decreases in ZBTB20 protein expression. This effect is mediated through upregulation of CUX1, as CUX1 silencing in miR122-silenced cells was shown to lead to both recovery of ZBTB20 levels and reduced AFP expression. Furthermore, the increased expression level of ZBTB20 in CUX1 knockdown cells suggests that ZBTB20 expression is regulated by CUX1. This miR122/CUX1/miR214/ZBTB20/AFP pathway may explain the deregulated AFP expression observed in HCC cells. Additionally, the ability of CUX1 to activate RhoA and to regulate the expression of many proteins involved in cell motility may explain the increased migration and invasiveness associated with malignancy of HCC [31] , [32] , [33] , [34] , [35] , [36] . It should be noted that, although this analysis revealed a trend toward inverse correlation between expression of miR122 and expression of AFP, this correlation could not be applied to all cases examined. Therefore, the possibility of additional pathways that regulate AFP expression cannot be discounted. Nonetheless, our results demonstrate that a decrease in miR122 function is a key factor that contributes to the regulation of AFP expression in HCC. MiR122 is the most abundant miRNA in the normal adult liver, comprising approximately 80% of all miRNAs [18] . The numerous reported roles of miR122 include regulation of cholesterol biosynthesis [19] , [20] , hepatitis C virus replication [49] and maintenance of the adult liver phenotype [21] . Specific miRNAs are often involved in the differentiation of specific cells and tissues [50] . As miR122 is liver-specific, we reasoned that this miRNA may have a role in the differentiation of normal hepatocytes. In our study, transgenic mice in which miR122 was functionally silenced were found to exhibit elevated AFP levels, but did not display abnormal morphological development in the liver (at least, not up to the age of 12 weeks), suggesting that decreased miR122 expression itself does not cause cells to become transformed. Ongoing characterization of these mice will be required to fully determine the physiological roles of miR122 in the noncancerous liver in vivo . In summary, we have shown that decreased miR122 expression in HCC is linked both to more biologically aggressive tumour behaviour and elevated AFP expression. Furthermore, both of these effects were shown to be mediated by increased expression of CUX1, a direct target of miR122. Similar strategies could also be used to develop new therapeutics and diagnostics for other cancers in which miRNAs that regulate both tumour characteristics and serum markers have been identified. Cell culture The human HCC cell lines, Huh7, PLC/PRF/5, HepG2, Hep3B and Huh1 were obtained from the Japanese Collection of Research Bioresources. The human embryonic kidney cell line, 293T and the human breast cancer cell line HS578T were obtained from the American Type Culture Collection . All cells were maintained in Dulbecco's modified Eagle medium, supplemented with 10% fetal bovine serum. Mouse experiments All experiments were carried out in compliance with the regulations of the Animal Use Committee of The University of Tokyo and The Institute for Adult Disease, Asahi Life Foundation. Generation of transgenic mice in which miR122 was functionally silenced Mice in which miR122 function was knocked down were generated using previously described protocols [38] , [51] . Briefly, a DNA fragment of 1,085 bp, containing the H1 promoter region, the coding region for the antisense miR122 stem-loop-stem RNA precursor, and a transcriptional terminator of five thymidines, was resected from the miRZip-122 construct described above by digestion with Pvu II. Proper silencing function of the resulting DNA was confirmed via transient transfection-based reporter assays that showed efficient knockdown of miR122 function. Stable C57BL/6 embryonic stem cell lines were generated by electroporation of the linearized transgene, and the resulting cells were injected into blastocysts by the UNITECH Company. Genotyping was performed by PCR using DNA isolated from tail snips. Four different mouse lines were maintained and the male littermates were used in experiments. Chromatin immunoprecipitation assay ChIP for CUX1 was performed as previously described [52] . For the scanning ChIP of the miR214 locus, realtime PCR analysis was performed using primer pairs specific for different regions of the promoters. Templates for the PCR reactions were 0.1% total input DNA (I), nonspecific DNA from sepharose beads alone (S), or chipped chromatin. The respective fold enrichment of the different DNA fragments are indicated relative to the DNA obtained by purification on sepharose beads without IgG (S). Enrichment was calculated using the HPRT locus as a reference. Doxycyclin-induced shRNA against CUX1 system For conditional knockdown of CUX1 in Hs578t cells, we took advantage of the Addgene plasmid 11643. HS578T cells were infected with pLVCT shCUX1(5,326–5,348)-tTRKRAB lentivirus as described [53] . At 48 h after infection, cells were split and cultured with or without doxycyclin at a final concentration of 2.5 μg ml −1 . Cells were used for experiments after 5 days of treatment. Doxycyclin was then removed from the culture media and cells were maintained for 4 days following release. Cell proliferation assay Relative cell proliferation was assessed using a Cell Counting Kit-8 (Dojindo Laboratories), as described previously [54] . Enzyme-linked immunosorbent assay AFP levels in the cell-culture supernatant were examined using an AFP-specific ELISA kit supplied by an outsourcing company, SRL. Western blot analysis Protein lysates were prepared from cells or mouse liver for immunoblot analysis. Proteins were separated by SDS–polyacrylamide gel electrophoresis and transferred to polyvinylidene difluoride membranes. After blocking with 5% dry milk to decrease nonspecific binding, membranes were probed with the appropriate primary antibodies. Primary antibodies were obtained from Abcam (ZBTB20, #ab48889, 1:500) and Santa Cruz Biotechnology (CDP, #sc-13024, 1:1,000). CUX1 antibodies (#861, 1:1,000) were generated as described previously [52] . Horseradish peroxidase-conjugated secondary antibodies were used to detect primary antibodies. Bound antibodies were detected using ECL Plus Western blotting detection reagents (GE Healthcare Life Sciences). Scratch assay The effects of miR122 knockdown on cellular migratory function were determined by evaluating cellular migration after scratching of a confluent monolayer of cells. Monolayers were cultured on 10 μg ml −1 fibronectin-coated dishes and were scratched using a 200-μl pipette. Migration was analysed at the indicated time points after scratching. In vitro invasion assay The effect of miR122 knockdown on invasive function was determined using BD BioCoat Matrigel Invasion Chambers (Becton Dickinson) according to the manufacturer's recommended protocol. Cell invasion was induced by removing the serum in the upper chamber. The number of invading cells was analysed after 22-h incubation. Cell numbers were counted in four randomly chosen fields at each time point. Quantitative pseudopodia assay Pseudopodium quantitation was performed using a Quantitative Pseudopodia Assay Kit (Chemicon) according to the manufacturer's instructions. Briefly, the upper chamber was coated with fibronectin and seeded with cells in serum-free medium. Serum was added to the lower chambers. 8 h later, pseudopodia on the lower surface were stained and eluted, and the absorbances of solubilized samples at 600 nm was measured using a microplate reader. CUX1-knockdown lentiviral construct Lentiviral particles expressing CUX1 shRNA were purchased from Santa Cruz Biotechnology (#sc-35051-V). In situ hybridization to assess miR122 and miR214 The expression of miR122 and miR214 in mouse liver and human HCC tissues was examined by in situ hybridization [55] , [56] . Locked nucleic acid (LNA)-scramble (negative control) and LNA-anti-miR122 and LNA-anti-miR214 probes were obtained from EXIQON. After deparaffinization, tissue sections were treated with 10 μg ml −1 proteinase K for 5 min at 37 °C and refixed with 4% paraformaldehyde, followed by acetylation with 0.25% anhydrous acetic acid in 0.1 M Tris–HCl buffer (pH 8.0). Following pre-hybridization for 30 min at 48 °C, hybridization was performed overnight with each 20 nM LNA probe in hybridization buffer (5xSSC buffer, 50% formamide, 500 μg ml −1 tRNA, 50 μg ml −1 Cot-1 DNA). After completion of hybridization, the sections were washed with 0.1×SSC buffer for 10 min at 52 °C three times and blocked with DIG blocking buffer (Roche Diagnostics) for 30 min. Sections were then probed with anti-DIG (1:500; Roche Diagnostics) for 1 h at room temperature. Detection was performed by incubation in NBT/BCIP buffer (Promega) overnight. Nuclei were stained with Nuclear FastRed (Sigma-Aldrich). Immunohistochemistry Tissue arrays containing HCC tissues were purchased from US Biomax. To determine the correlations between AFP, ZBTB20, CUX1, miR122 and miR214 expression and HCC differentiation grade, slides carrying consecutive sections were obtained. Slides were baked at 65 °C for 1 h and deparaffinized. Endogenous peroxidase activity was blocked by incubation in 3% hydrogen peroxide buffer for 30 min. Antigen retrieval was performed by incubating the slides at 89 °C in 10 mM sodium citrate buffer (pH 6.0) for 30 min. To minimize nonspecific background staining, slides were blocked in 5% normal goat serum (Dako) for 10 min at room temperature. Tissues were labelled overnight at 4 °C with primary antibodies raised against AFP (Dako, #N1501, 1:100), CUX1 (#sc-13024, 1:100) and ZBTB20 (HPA016815, Sigma-Aldrich, 1:100). Slides were then incubated with anti-rabbit horseradish peroxidase-conjugated secondary antibodies (Nichirei Bioscience) for 1 h. Primary antibody binding was visualized by incubation in 3,3′-diaminobenzidine in buffered substrate (Nichirei Bioscience) for 5 min. The slides were counterstained with haematoxylin, dehydrated with ethanol, and mounted with Clarion mounting medium (Biomeda). GTP-binding RhoA and Rac1 immunoprecipitation assay The amount of RhoA activity was examined using an Active Rho Pull-down and Detection Kit (Thermo Fisher Scientific) according to the manufacturer's recommended protocol. The amount of GTP-bound RhoA protein (the active form of RhoA) was detected by Western blotting with the provided anti-RhoA antibody (1:100). Rac1 activity was similarly determined by using PAK-GST Protein Beads (#PAK02, Cytoskeleton) for pulldowns and anti-Rac1 antibodies (1:100) for subsequent Western blotting (#89856D, Thermo Fisher Scientific). Orthotopic xenograft tumour model of HCC Male BALB/c (nu/nu) nude mice were purchased from CREA Japan (Tokyo, Japan). The transplantation of tumour cells into mouse livers was performed using previously reported methods [57] , [58] . Briefly, 2×10 6 control or miR122-silenced PLC/PRF5 cells were suspended in 30 μl of PBS containing 1% Matrigel (Becton Dickinson). After anaesthesia, the liver was exposed through a surgical incision. Cells were slowly injected under the capsule of left lobe of the liver using a 28-gauge needle. When successful, a transparent bleb of cells could be seen through the liver capsule. After injection, light pressure was applied to the injection site with sterile gauze for 2 min to prevent bleeding and tumour cell leakage. The abdomen was then closed with sutures. Transplantation was successful in a total of 12 mice (6/group). At 4 weeks post-transplantation, liver tissues were collected, serially sectioned, and stained with haematoxylin and eosin. Statistical analysis Statistically significant differences between groups were determined using Student's t -test when variances were equal. When variances were unequal, Welch's t -test was used instead. P -values less than 0.05 were considered statistically significant. Plasmid and stable cell line construction, reporter assays, RT–PCR, northern blotting and immunocytochemistry are described in the Supplementary Methods . All primer information is provided in Supplementary Table S1 . How to cite this article: Kojima, K. et al . MiRNA122 is a key regulator of α-fetoprotein expression and influences the aggressiveness of hepatocellular carcinoma. Nat. Commun. 2:338 doi: 10.1038/ncomms1345 (2011).